Janus graphene from asymmetric two-dimensional chemistry Janus materials have distinct surfaces on their opposite faces. Graphene, a two-dimensional giant molecule, provides an excellent candidate to fabricate the thinnest Janus discs and study the asymmetric chemistry of atomic-thick nanomembranes using covalent chemical functionalisation. Here we present the first experimental realisation of nonsymmetrically modified single-layer graphene—Janus graphene—which is fabricated by a two-step surface covalent functionalisation assisted by a poly(methyl methacrylate)-mediated transfer approach. Four types of Janus graphene are produced by co-grafting of halogen and aryl/oxygen-functional groups on each side. Chemical decorations on one side are found to be capable of affecting both chemical reactivity and physical wettability of the opposite side, indicative of communication between the two grafted groups. This novel asymmetric structure provides a platform for theoretical and experimental studies of two-dimensional chemistry and graphene devices with multiple functions. Janus nanostructures have attracted much attention in recent years, with potential applications as novel sensors, actuators and surfactants, because of their remarkably interesting surface activities [1] , [2] , [3] . For instance, the two-dimensional (2D) Janus disc has a remarkable stabilisation effect for the oil-water interface [4] , drawing interest in the applicability of Janus nanostructures as a novel class of future surfactant. It is noted that the synthesis of 2D Janus nanostructures depends critically on the fabrication of extremely thin but mechanically stable and self-supporting 2D nanomaterials. Graphene, a one-atom-thick hexagonal mesh of carbon atoms, has stimulated enormous interest as a new member of the carbon allotrope family and provides new opportunities for the fabrication of 2D Janus discs [5] . For graphene, the extremely high carrier mobility, mechanical flexibility, optical transparency and versatility for band structure engineering make it a promising candidate for post-silicon electronics [6] , [7] , [8] . Although the physical properties of graphene have been at the centre of attention, graphene chemistry—the functionalisation of graphene as a 2D giant molecule—offers a new direction to tailor its optical, electronic and surface properties, through the introduction of variable chemical decorations [9] , [10] , [11] . Physisorption of chemical species on graphene would provide a facile way to alter its electronic properties [12] , however, covalent chemical modification shows a great advantage in achieving permanent stabilisation for long-term usage [13] . Previous attempts towards fundamental research on covalent functionalisation of graphene mainly involved the development of new modification strategies (for example, hydrogenation [14] , [15] , [16] , [17] , fluorination [18] , [19] , [20] , chlorination [21] , [22] , diazotization [23] , [24] , [25] , [26] , [27] and other cycloaddition reactions [28] , [29] , [30] , [31] ), covalent addition of edge and defects [27] , [32] , fabrication of chemical superlattices [26] , [33] and quantum effects in graphene modification [17] , [34] . Of the various significant research activities on graphene chemistry that have been conducted, nearly no work to date has been focused on the asymmetric chemistry of this ideal 2D atomic crystal via covalently attaching different functional groups on its two faces simultaneously. Graphene is composed of carbon atoms that are held together by strong covalent bonds, which are theoretically predicted [35] and experimentally confirmed [36] , [37] , [38] , [39] , [40] to be impermeable to small atoms and molecules as a perfect nanoballoon at room temperature. This is a prerequisite for its bifacially nonsymmetrical modification. Previous works have shown that free-standing graphene exhibits higher chemical functionalisation extent at the same condition in comparison with graphene supported by a substrate, because only one side of the latter is accessible to the reactants [14] , [18] . This unique property, as well as the availability of various approaches towards graphene functionalisation, allows us to further develop a facile approach to engineering graphene nonsymmetrically, by attaching its two sides with different functionalities. In addition, nonsymmetrical modification exhibits an advantage in modifying the bandgap of graphene. Our recent theoretical work has proven that the nonsymmetrical functionalisation breaks the symmetric restrictions of graphene, giving it a robust non-zero gap, which is nearly linearly correlated with the binding energy difference between the two functionalities. In this paper, we experimentally demonstrate a new functional graphene derivative—Janus graphene—which comprises two types of functional groups separated by the single-mediated carbon layer (described as X-G-Y), as Fig. 1 illustrates. Our strategy in fabrication is based on the utilisation of poly(methyl methacrylate) (PMMA) film with typical thickness of 200–300 nm as a flexible macroscopic mediator for a two-step functionalisation. Using photochlorination, fluorination, phenylation, diazotization and oxygenation reactions, four types of Janus graphene have been obtained by cografting X (halogen groups) and Y (aryl or oxygen-functional groups) on each side. More importantly, we observed that the functionalities on one side are capable of influencing the chemical reactivity as well as surface wettability of the opposite side, indicative of a communication between X and Y through the mediated single carbon layer. Such novel structures would offer an excellent alternative to study asymmetric chemistry of graphene, control the self-assembly of graphene-based new functional structures [41] and advance the potential applications of graphene functional derivatives as a 2D sensor or actuator for biochemical detection [33] , [38] , [39] , [40] . 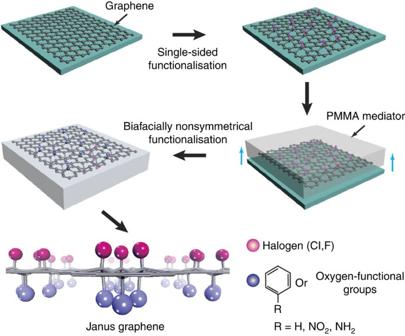Figure 1: Schematic illustration of the poly(methyl methacrylate) (PMMA)-mediated transfer procedure to fabricate Janus graphene. Spin-coating a PMMA film on the single-sided functionalised graphene layer, peeling off PMMA/graphene from the substrate, turning over to nonsymmetrically modify the other side of graphene with the protection of PMMA as the substrate and finally removing the PMMA to obtain Janus graphene. Figure 1: Schematic illustration of the poly(methyl methacrylate) (PMMA)-mediated transfer procedure to fabricate Janus graphene. Spin-coating a PMMA film on the single-sided functionalised graphene layer, peeling off PMMA/graphene from the substrate, turning over to nonsymmetrically modify the other side of graphene with the protection of PMMA as the substrate and finally removing the PMMA to obtain Janus graphene. Full size image Fabrication of Janus graphene Two types of monolayer graphene samples were employed: graphene flakes mechanically exfoliated from Kish graphite and graphene films grown by chemical vapour deposition (CVD) on copper foils. The CVD-grown graphene was detached by etching the copper away with 2.0 M Fe 2 (SO 4 ) 3 aqueous solution and transferred onto 300 nm silicon oxide/silicon (SiO 2 /Si) substrate. Single-layer mechanical exfoliated graphene was located by optical microscopy and subsequently identified via Raman spectroscopy. 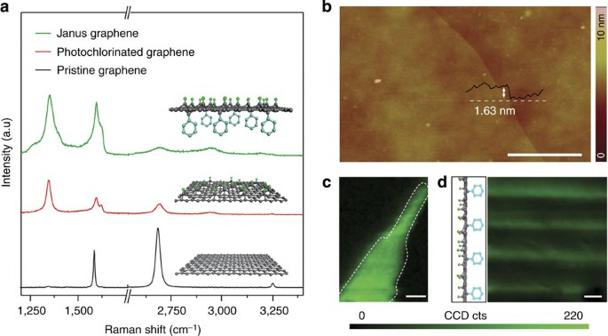Figure 2: Raman and AFM characterisation of Janus graphene cografted with chlorine and phenyl groups on the opposite side. (a) Raman spectra (λex=514.5 nm) evolution in the fabrication process of Janus graphene and the insets show schematic illustrations. (b) Typical AFM image of exfoliated monolayer graphene after the nonsymmetrical modification of phenyl and chlorine groups. The height profile is taken along the dotted line, representing the intact film structure. Scale bar, 1 μm. (c) Intensity map of the D band for Janus graphene, demonstrating the uniform distribution of the chemical decorations. The white dotted curve shows the position of the graphene flake. Scale bar, 5 μm. (d) D-band mapping for a patterned Janus graphene structure, which is illustrated schematically on the left. Scale bar, 5 μm. Figure 2a demonstrates the evolution of Raman spectrum in the fabrication process of Janus graphene. Single-sided photochlorination of individually exfoliated monolayer graphene was first carried out on 300 nm SiO 2 /Si, following the procedures described by our group previously [21] . Chlorine molecules were introduced to our home-made quartz reaction vessel by air-flow carrying a chlorine/nitrogen mixture under 1 atm of pressure. A xenon lamp with wavelength of 250–450 nm and maximum power intensity of 0.9 W cm −2 was employed to initiate chlorine molecules to split into highly reactive chlorine radicals, which were consequently combined with graphene by a free radical addition reaction. Raman disorder-induced mode (D band at 1,330 cm −1 ) of graphene emerges and increases ( Supplementary Fig. S1 ) with irradiation time, indicative of the transformation of carbon network from sp 2 to sp 3 configurations [42] . As shown in Fig. 2a , nearly no D band was observed in pristine monolayer graphene, and G′ band (2,687 cm −1 ) is about three times more intense than G band (1,587 cm −1 ). After single-sided photochlorination, a pronounced D band as well as an extra D′ band (1,620 cm −1 ) was detected, while the G′ band was suppressed dramatically owing to the chemical doping effect [43] . Formation of covalent C–Cl bonds, confirmed by X-ray photoelectron spectroscopy (XPS) measurements ( Supplementary Fig. S2 ), gave rise to the blue shift of G (from 1,587.5 to 1,595.0 cm −1 ) and G′ peaks (from 2687.4 to 2,691.2 cm −1 ) in the Raman spectrum ( Fig. 2a ), consistent with the strong electron-drawing capability of chlorine as suggested by our previous calculations [44] . Figure 2: Raman and AFM characterisation of Janus graphene cografted with chlorine and phenyl groups on the opposite side. ( a ) Raman spectra ( λ ex =514.5 nm) evolution in the fabrication process of Janus graphene and the insets show schematic illustrations. ( b ) Typical AFM image of exfoliated monolayer graphene after the nonsymmetrical modification of phenyl and chlorine groups. The height profile is taken along the dotted line, representing the intact film structure. Scale bar, 1 μm. ( c ) Intensity map of the D band for Janus graphene, demonstrating the uniform distribution of the chemical decorations. The white dotted curve shows the position of the graphene flake. Scale bar, 5 μm. ( d ) D-band mapping for a patterned Janus graphene structure, which is illustrated schematically on the left. Scale bar, 5 μm. Full size image The key step in fabricating Janus graphene is to expose the fresh side, which was protected by the substrate in the first modification process, for the next nonsymmetrical functionalisation. A PMMA film was used as a flexible mediator to peel off the single-sided chlorinated graphene from the substrate nondestructively in a 2% HF aqueous solution at room temperature. Phenylation of graphene [45] was performed subsequently on the exposed side to fabricate Janus graphene. After adsorbing a uniform thin layer of benzoyl peroxide (BPO) molecules ( Supplementary Fig. S3 ), the mediator was subject to an extended laser irradiation ( λ ex =514.5 nm, 0.5 mW) with graphene facing up to the laser. A more pronounced increase in the D band ( Fig. 2a ) in comparison with that of the previous single-sided photochlorinated graphene suggests its further functionalisation by attaching phenyl groups on the opposite side of chlorine. Either G band (from 1,595.0 to 1,594.2 cm −1 ) or G′ band (from 2,691.2 to 2,691.0 cm −1 ) shift in the Raman spectrum was observed after phenylation, which is consistent with the weak electron-drawing capability of grafted phenyl groups, as predicted by theoretical calculations [46] . This observation can also exclude possible photo-oxidation in the phenylation process, as oxygen species always introduce a strong p-doping effect to carbon systems [47] . To release Janus graphene, the mediator was attached onto the target substrate with Janus graphene facing down to the substrate and dissolved in acetone vapour. The atomic force microscopy (AFM) image of Janus graphene exhibits a continuous film ( Fig. 2b ), indicating that the two-step covalent addition would not destroy the physical intactness of the carbon bonds. The nondestructive nature of carbon domains can also be confirmed by the high-resolution transmission electron microscopy (TEM) and selected area electron diffraction (SAED) images ( Supplementary Fig. S4 ). Statistical AFM measurements ( Supplementary Fig. S5 ) show the height of Janus graphene is in the range of 1.2–2.0 nm with an average at 1.6 nm, slightly larger by a value of 0.6 nm than the height of pristine graphene, which is in the range of 0.7–1.2 nm (with an average at 1.0 nm). We interpret the increase in height as being a result of the addition of phenyl and chlorine groups as well as the corrugation induced by the covalent addition. The D band intensity of Janus graphene in the Raman spectrum was recorded as a 2D map ( Fig. 2c ). The homogenous colour distribution in a large area scan suggests the uniformity of functionalisation in Janus graphene within the spatial resolution of Raman instruments (~1 μm). In addition, it is notable that using a laser spot as the light source to initiate the phenylation controlled patterning can be easily achieved by ‘direct-writing’, which facilities the fabrication of Janus graphene superlattices. As shown in Fig. 2d , a Janus graphene superlattice structure can be easily visualised in a Raman D band intensity map. A more pronounced D band was detected in the regions that the laser passed by (green) relative to the others (dark), suggesting further functionalisation by attaching phenyl groups. Such controllable localised attachment in the Janus graphene superlattice may provide great versatility for creating graphene-based chemical sensors and other electronic devices [33] . Other types of Janus graphene In principle, arbitrary pairs of functionalities can be attached onto the opposite sides of graphene to create various kinds of Janus graphene. For instance, fluorination and oxygenation reactions could be combined together to create Janus graphene of fluorine-graphene-oxygen [19] , [48] . XPS survey, the evolution of Raman spectra, and surface wettability measurements confirm that the fluorine and oxygen groups were cografted successfully ( Supplementary Figs S6,S7 ). Here, we show another example by using diazotization of graphene in the second step of functionalisation, in view of its simplicity and versatility [23] , [24] , [25] , [27] . Peeled mediator embedding chlorinated graphene was submerged into ~20 mM diazonium salt (4-nitrobenzene diazonium tetrafluoroborate) aqueous solution for 1–2 h at 40 o C without stirring, allowing only the exposed surface to react and undergo surface functionalisation to form covalently bonded aryl-substituents. An increase of D band in Raman spectrum ( Supplementary Fig. S8 ) with respect to the single-sided chlorinated graphene suggests a higher extent of functionalisation resulting from the covalent attachment of nitro phenyl groups on the opposite of chlorine. The XPS survey spectrum ( Fig. 3a ) reveals N1s and Cl2p peaks both in Janus graphene. The high-resolution N1s spectrum shows an additional pronounced peak ( Fig. 3b and Supplementary Fig. S9 ) centred at 406.2 eV (labelled by * and assigned to nitro groups [23] , [24] ), confirming the presence of nitro phenyl groups on Janus graphene. The lower N1s peaks is associated with the presence of reduced nitrogen species introduced by the transferring procedure and may be due to transformation of the nitro groups by X-ray irradiation in the XPS spectrometer chamber [49] . It is notable that the decorations on each side could offer useful platforms for further chemical functionalisation. For instance, the nitro groups can be chemically reduced, providing an alternative way to fabricate new types of Janus graphene. In the experiment, 5 g reduced ion powder was added into a mixture of 0.5 ml HCl, 10 ml deionised (DI) water and 4 ml isopropanol to generate reactive hydrogen species in the durative reduction. The recorded XPS N1s spectra ( Fig. 3b ) showed a single peak centred at 399.2 eV after 5 h reduction, assigned to the amino group nitrogen [24] . The reduction of surface functionalities was also confirmed by the evolution of surface wettability ( Supplementary Fig. S10 ). 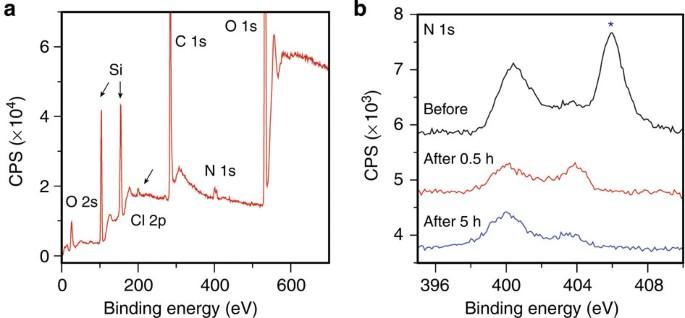Figure 3: XPS spectra of Janus graphene cografted on opposite sides with chlorine and nitro phenyl groups. (a) The low resolution survey measured on 300 nm SiO2, in which the surface coverage of nitro phenyl and Cl groups was approximated at 2.1% and 0.8%, respectively. (b) N1s core level spectrum, showing the XPS spectrum evolution with the reduction time. The blue label (*) indicates the nitro-group signal. Figure 3: XPS spectra of Janus graphene cografted on opposite sides with chlorine and nitro phenyl groups. ( a ) The low resolution survey measured on 300 nm SiO 2 , in which the surface coverage of nitro phenyl and Cl groups was approximated at 2.1% and 0.8%, respectively. ( b ) N1s core level spectrum, showing the XPS spectrum evolution with the reduction time. The blue label (*) indicates the nitro-group signal. Full size image Monolayer graphene is an atomic-thick nanomembrane, providing an ideal platform to theoretically and experimentally study the interaction between nonsymmetrically modified functionalities on a molecular level. The band structure of Janus graphene was first considered from a theoretical point of view. Janus-type engineering of graphene (Cl-G-phenyl) is superior to symmetrical functionalisation (Cl-G-Cl and phenyl-G-phenyl) on the bandgap modulation at the same coverage of decorations ( Supplementary Fig. S11 ). Experimentally, we employed Raman spectroscopy to understand the influence of chlorine groups on the kinetics of phenylation on the opposite side, considering the term I D / I G is usually used to describe the modification extent under certain circumstance [50] . 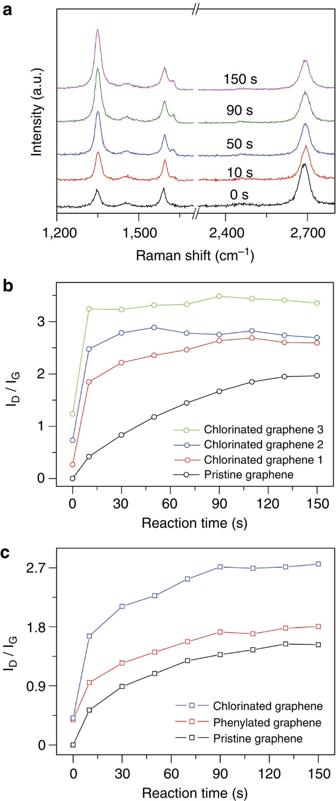Figure 4: The influences of functionalities to the kinetics of phenylation on the opposite side. (a)In situRaman spectra of chlorinated graphene during the phenylation process on the opposite side of the chlorine groups. Change ofID/IGin response to the phenylation time under different initial chlorination extent (b) and varied functionalities (c) on the opposite side. Figure 4a shows the time evolution of the Raman spectrum for chlorinated monolayer graphene after a series of phenylation reactions. The D band grows in intensity essentially linearly, without a significant change in its width or shape, indicative of the increase of chemical decorations on the opposite side. In addition, the I D / I G will become saturated at a certain value, suggesting the adsorbed BPO molecules have been completely consumed. To examine the influence of the opposite chlorine groups, we carried out the phenylation reaction on chlorinated monolayer graphene with varied decoration extent. As seen from Fig. 4b , the reaction rate, indicated by the slope of I D / I G versus phenylation time curve, increased monotonically together with the increase of chlorination extent, especially at the first few tens of seconds. More importantly, even a little decoration of chlorine groups can dramatically affect the kinetics of phenylation, leading to a rapid increase in I D / I G . Previous work has shown that grafted functionalities would introduce a noticeable geometric distortion with a characteristic radius of 5 Å and lead to a sharp decrease of reaction potential barriers in these regions, similar to the case of graphene with defects [51] . This can well explain the dramatic increase in the phenylation rate even with a little chlorine decoration. Figure 4: The influences of functionalities to the kinetics of phenylation on the opposite side. ( a ) In situ Raman spectra of chlorinated graphene during the phenylation process on the opposite side of the chlorine groups. Change of I D / I G in response to the phenylation time under different initial chlorination extent ( b ) and varied functionalities ( c ) on the opposite side. Full size image The influence of different groups on the opposite-sided phenylation was also examined, and the results are summarised in Fig. 4c . A particularly interesting phenomena is that no discernible change in phenylation kinetics was detected when having phenyl groups (at I D / I G =0.2) on the opposite side relative to the pristine graphene, indicating that a little decoration of phenyl groups would not increase the phenylation rate of the opposite side until a large modification extent ( Supplementary Fig. S12 ). In contrast, phenylation with the same decoration extent of chlorine groups on the opposite side led to a rapid increase of I D / I G , dramatically changing the phenylation kinetics. From our previous calculations [44] , chlorine groups are covalently bonded onto graphene in the form of pairs at the initial stage, and with increasing chlorine coverage, this configuration may further cluster into hexagonal rings. On the contrary, the phenyl groups on graphene will prefer to distribute randomly in view of its steric hindrance [46] . We believe it is this cluster configuration of chlorine groups that introduces a greater activation effect to the phenylation on the opposite side, thus leading to a dramatic increase in the reaction rate. Graphene is a one atomic thick hexagonal mesh of carbon atoms, providing an excellent candidate to fabricate the extremely thin but mechanically stable and self-supporting Janus nanostructure. Through nonsymmetrically bifacial cografting of different functionalities on the opposite sides, Janus graphene is supposed to exhibit anisotropic surface wettability, providing a novel potential one atom thick surfactant structure. We performed static water contact angle measurements to monitor the surface wettability evolution of the two sides during Janus graphene fabrication. In the control experiment, no discernible contact angle difference was observed on the two sides of graphene without any chemical treatment ( Supplementary Fig. S13 ). 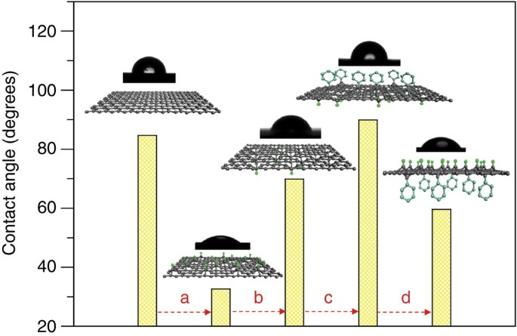Figure 5: The functional graphene derivative with bifacially anisotropic wettability. Static water contact angle measurements in the fabrication procedures of Janus graphene: (a) single-sided photochlorination; (b) exposure of graphene fresh side; (c) single-sided phenylation; (d) release of Janus graphene. The insets exhibit images of water droplets and schematic illustrations of the related surfaces. Figure 5 typically exhibits the contact angle evolution of one sample during the Janus graphene fabrication. Single-sided chlorination results in a decrease in the contact angle, from 84.7 ° to 32.6 ° as recorded, owing to the formation of C–Cl bonds, which would increase surface energy and simultaneously introduce polarity. The contact angle of the opposite side, however, slightly dropped to 69.9 ° , indicating that the chlorine groups are capable of influencing the wettability of the opposite side (more results are shown in Supplementary Fig. S14 ). Phenylation results in reduced wettability of the exposed surface and the contact angle increased to 89.9 ° after introducing the phenyl groups. Meanwhile, the contact angle of the chlorinated side also increased from 32.6 ° to 59.6 ° as recorded. The difference of contact angles on the two sides can reach as high as 30 ° (89.9 ° on the phenylated side while 59.6 ° on the chlorinated side). Thus, we can draw the conclusion that when cografting different chemical decorations on the opposite side of graphene, the surface wettability of the two sides can influence each other. We believe these influences originate from the extreme thinness of the medium single carbon layer [52] and the polarity introduced by the formation of covalent bonds. Figure 5: The functional graphene derivative with bifacially anisotropic wettability. Static water contact angle measurements in the fabrication procedures of Janus graphene: ( a ) single-sided photochlorination; ( b ) exposure of graphene fresh side; ( c ) single-sided phenylation; ( d ) release of Janus graphene. The insets exhibit images of water droplets and schematic illustrations of the related surfaces. Full size image In summary, we demonstrated a universal route to fabricate a nonsymmetrically modified graphene derivative called Janus graphene with distinct and different functionalities on its sides. This atomically thick sheet provides an ideal 2D bifacial Janus system to study asymmetric chemistry as the decorations on each side offer useful platforms for further chemical functionalisation. In view of the extreme thinness of the medium single carbon layer, chemical functionalities on one side are capable of affecting both chemical reactivity and surface wettability of the opposite side, indicative of communication between the two grafted groups through the mediated carbon layer. This novel graphene nonsymmetric structure makes 2D graphene devices with various functionalities conceivable. Preparation of graphene samples Two types of monolayer graphene samples were employed in this work: graphene flakes mechanically exfoliated from Kish graphite and graphene films grown by CVD on copper foils, respectively. Single-layer mechanical exfoliated graphene were located and identified by optical microscope (Olympus DX51, Olympus) and Raman spectrum (Horiba HR800, 514.5 nm excitation wavelength). CVD growth of graphene on copper foil was carried out at temperatures up to 1,000 °C by CVD using a mixture of 35 sccm CH 4 and 2 sccm H 2 at a total pressure of 500 mTorr. The as-grown graphene films are predominately monolayer, with a small percentage (less than ~5%) of the area having few layers, owing to the self-limiting effect of copper surface under low growth pressure. To avoid the precontamination of Cl species, the CVD-grown graphene was detached by etching the copper away with 2.0 M Fe 2 (SO4) 3 aqueous solution rather than FeCl 3 as our previous work reported [21] . Functionalisation of graphene Photochlorination of graphene was conducted in a home-made gas-phase reaction system following the procedures our group developed previously [21] . Chlorine gas was obtained by adding 15 ml hydrochloric acid 9 M slowly into 5 g MnO 2 at 60 o C and dried by concentrated sulphuric acid before entering the photoreactor (6 × 3 × 2.5 cm 3 ; transmittance is >85% in the UV zone). A xenon lamp (PLS-3SXE300W) with a maximum power density of 0.9 W cm −2 was employed as the light source of the photochlorination reaction, in which long wavelength (>450 nm) light was filtered out. The photochlorination was performed under an atmosphere of dry nitrogen with the rigid exclusion of air and moisture by using standard Schlenk technique. Fluorination was performed in a Teflon container at the temperature of 40 o C in a glove box, in which the O 2 concentration is <6 ppm and H 2 O is <5 ppm Graphene grown on copper foil was exposed to atomic F formed by decomposition of xenon difluoride (XeF 2 ). This approach is superior to the possible fluorination in F 2 plasma as the use of XeF 2 avoids a potential damage as a result of the ion bombardment. After fluorination, each sample was rinsed copiously with NaOH (10 wt %) and DI water to ensure the removal of residual XeF 2 reagent on the surface. Phenylation of graphene was conducted under the irradiation of Raman laser (Horiba HR800, 514.5 nm excitation wavelength) with the power density of ~2 mW. The laser spot size is about 1 μm. A uniform thin layer of BPO molecules was adsorbed by submerging graphene into a 0.5 mM BPO isopropanol solution for 0.5 h, where isopropanol was chosen as the solvent owing to its compatibility with PMMA. To achieve a large area of homogenous phenylation, Raman mapping was conducted by piezo-driving mirror scanning with a step size of 0.5 μm. The integration time during mapping was 0.7 s. After phenylation, the mediator embedding Janus graphene was submerged into isopropanol for >1 h in order to remove the residual BPO molecules adsorbed. Diazotization of graphene was conducted following the procedures described previously [27] . Two millilitre 1 wt % anionic surfactant SDS aqueous solution was added into 10 ml 20 mM diazonium salt (4-nitrobenzene diazonium tetrafluoroborate) aqueous solution to form the reactant solution, in which the peeled mediator embedding chlorinated graphene was submerged into for 1–2 h at 40 o C without stirring, allowing only the exposed surface to react and undergo surface functionalisation to form covalent bonded aryl-substituents. After reaction, each sample was rinsed copiously with DI water and immersed for an additional 2 h to ensure the removal of residual diazonium reagent on the surface. Fabrication of Janus Graphene After the single-sided halogenation, a PMMA solution (M W =950 K, 4 wt%, AR-P679.04, Allresist) was spin-coated (2,000 r min −1 , 1 min) onto the single-sided functionalised graphene and baked at 170 o C for 5 min to obtain a mediator embedding halogenated graphene. The peel off process was achieved in a 2% HF aqueous solution at room temperature (~15 min) to separate the mediator from the substrate and expose the opposite side of graphene simultaneously. The PMMA/graphene film can be easily manipulated under the assistance of a scotch tape. After the second step functionalisation, PMMA/graphene was attached onto the target substrate with graphene side facing down to the target substrate. PMMA was removed by acetone vapour. Characterisation Raman spectroscopy (Horiba HR800) with laser excitation energy of 514.5 nm (2.41 eV) was used to evaluate the modification results. The laser spot size is about 1 μm. Raman mapping was conducted by piezo-driving mirror scanning with a step size of 0.5 μm. The integration time during mapping was 3 s. XPS measurements were carried out using a Kratos Axis Ultra spectrometer with Al ka monochromated X-ray at low pressures of 5 × 10 −9 to 1 × 10 −8 Torr. The large area CVD-grown single-layer graphene film was used for XPS characterisation. The collection area was about 300 × 700 μm 2 . The highest peak in C1s spectra was shift to 284.8 eV for charge correction. Atomic force microscope (Veeco Nanoscope IIIa) in tapping mode was used for morphology studies of Janus graphene sheets. Before AFM test, the sample was annealed up to 320 o C for 40 min in the mixture of 400 sccm Ar and 100 sccm H 2 to further remove the residues. TEM of Janus graphene was studied by a 200 kV FET Tecnai F20 TEM apparatus. The Janus graphene was detached by etching the supporting SiO 2 substrate away with a dilute HF aqueous solution (2 wt%) and subsequently transferred onto a copper grid with the assistance of PMMA film. The PMMA film was then removed with acetone. Static contact-angle measurements were conducted on OCA-20 by placing a droplet of DI water on the surface of graphene, and all the tests were performed in the air at room temperature. How to cite this article: Zhang, L. et al. Janus graphene from asymmetric two-dimensional chemistry. Nat. Commun. 4:1443 doi: 10.1038/ncomms2464 (2013).